Whole-exome sequencing identifies somaticATRXmutations in pheochromocytomas and paragangliomas Pheochromocytomas and paragangliomas (PCC/PGL) are the solid tumour type most commonly associated with an inherited susceptibility syndrome. However, very little is known about the somatic genetic changes leading to tumorigenesis or malignant transformation. Here we perform whole-exome sequencing on a discovery set of 21 PCC/PGL and identify somatic ATRX mutations in two SDHB -associated tumours. Targeted sequencing of a separate validation set of 103 PCC/PGL identifies somatic ATRX mutations in 12.6% of PCC/PGL. PCC/PGL with somatic ATRX mutations are associated with alternative lengthening of telomeres and clinically aggressive behaviour. This finding suggests that loss of ATRX, an SWI/SNF chromatin remodelling protein, is important in the development of clinically aggressive PCC/PGL. Pheochromocytomas and paragangliomas (PCC/PGL) are tumours of the autonomic nervous system arising from the adrenal medulla and extra-adrenal ganglia, respectively. PCC/PGL are more commonly associated with inherited susceptibility gene mutations than any other solid tumour. In fact, up to 40% of PCC/PGL have a germline mutation in one of twelve genes, which are known to be associated with an increased risk of PCC/PGL, including VHL, RET, NF1, SDHA, SDHB, SDHC, SDHD, SDHAF2, TMEM127, MAX, EPAS1 and FH [1] . However, very little is known about the somatic genetic or genomic changes leading to tumorigenesis or malignant transformation. Most studies have identified somatic mutation rates <5% for candidate genes tested in PCC/PGL [2] , [3] , [4] , [5] , [6] . Somatic HRAS mutations have been identified in 10% of sporadic PCC/PGL without a known inherited mutation [7] . Somatic mutations in known susceptibility genes such as NF1, VHL and RET are seen at rates between 5 and 40% depending on the gene and the study, and these somatic mutations are seen almost exclusively in sporadic PCC/PGL as well [8] , [9] , [10] , [11] . Somatic mutations in the SDHx genes are rarely, if ever, observed [9] , [12] , [13] , [14] . Most patients with PCC/PGL have clinically benign disease but a fraction have clinically aggressive tumours. Patients with benign PCC/PGL usually have a single tumour, but some have more aggressive disease and develop multiple primary tumours throughout their lifetime. Approximately one-fourth of patients with PCC/PGL have malignant disease defined by the presence of distant metastases [15] , and when metastatic, PCC/PGL are associated with a 50% 5-year survival rate [16] . Another group of patients have PCC/PGL with extensive local invasion or recurrence at the primary site, and although this group does not meet criteria of malignancy due to the absence of distant metastases, they share a similar burden of excessive catecholamine secretion, which is not easily surgically cured. Systemic treatments used for both malignant and clinical aggressive tumours have limited efficacy [17] . No reliable predictors of aggressive disease exist other than a germline mutation in the Succinate dehydrogenase (SDH) B gene, which confers a higher risk of malignancy (31–75%) than mutations in other susceptibility genes (usually <5%) [18] . Only half of patients with metastatic disease carry inherited SDHB mutations [19] , meaning many of the patients who develop malignant PCC/PGL had no known predictors of malignant potential. Thus, it is critically important to both identify molecular predictors of malignancy and new targets for therapeutic intervention. Here, we aim to identify driver mutations for clinically aggressive PCC/PGL by performing whole-exome sequencing (WES) on a discovery set of 21 fresh-frozen tumour/matched germline DNA samples. We identify two SDHB -associated tumours with somatic ATRX mutations. Using a separate validation set of DNA from 103 formalin-fixed paraffin-embedded (FFPE) PCC/PGL, we find somatic ATRX mutations in 12.6% of tumours. We are the first to report ATRX mutations in PCC/PGL and suggest that ATRX loss is important for tumorigenesis in a subset of PCC/PGL. Low number of somatic mutations in PCC/PGL We performed WES on a discovery set of 21 fresh-frozen tumour/matched germline DNA samples. Using Agilent SureSelect All Exon v3 technology for exome capture, the mean depth of coverage was 84 × in tumour DNA and 85 × in germline DNA. To identify somatic mutations, we removed any variant seen in the matched germline sample and followed a strict filtering algorithm for variant calling, including removing variants with MAF>0.1% in 1,000 genomes and/or ESP6500, with read depth <20 or segmental duplication >80%. 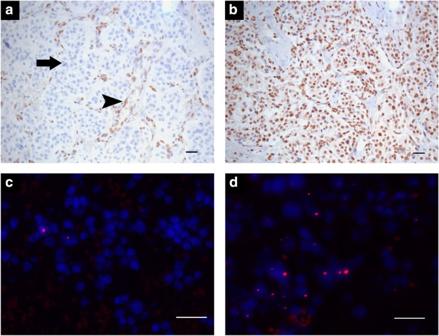Figure 1: Immunohistochemistry and immunofluorescence in PCC/PGL with somaticATRXmutations. FFPE tumour PP119Z1 shows absence of ATRX in tumour cells (arrow;a) with the presence in endothelial cells (arrow head) as an internal control; DAXX staining was positive (b). Telomere FISH shows alternative lengthening of telomeres in twoSDHB-associated PCC/PGL with somaticATRXmutations from the discovery and validation sets, PP119Z1 (c) and PP142Z1 (d), respectively. Scale bars, 30 μm. After removing synonymous variants, there was a mean of 17.38±6.27 somatic mutations per tumour ( Supplementary Table 1 ). This relatively low number of mutations in PCC/PGL is consistent with that seen in related tumour types, such as neuroblastomas (~12–18/tumour) and pancreatic neuroendocrine tumours (PNETs; ~16/tumour) [20] , [21] . We examined for somatic mutations in the known susceptibility genes. Consistent with the literature, we found that three of seven sporadic tumours had somatic mutations in NF1 . No somatic mutations were seen in other known common or rare susceptibility genes ( SDHx, TMEM127, RET, VHL, MAX, FH, EPAS1, KIF1B, EGLN1 or MEN1 ) in any tumours in the discovery set. Interestingly, two of seven SDHB -associated tumours had deleterious variants in ATRX (PP119F1 p.W2275X and PP098F2 p.R2197H in the conserved helicase domain at an amino-acid residue also reported to be altered in neuroblastoma [21] ) ( Supplementary Table 2 ). ATRX protein was absent in the tumour cells by immunohistochemistry (IHC) ( Fig. 1 ). Figure 1: Immunohistochemistry and immunofluorescence in PCC/PGL with somatic ATRX mutations. FFPE tumour PP119Z1 shows absence of ATRX in tumour cells (arrow; a ) with the presence in endothelial cells (arrow head) as an internal control; DAXX staining was positive ( b ). Telomere FISH shows alternative lengthening of telomeres in two SDHB -associated PCC/PGL with somatic ATRX mutations from the discovery and validation sets, PP119Z1 ( c ) and PP142Z1 ( d ), respectively. Scale bars, 30 μm. Full size image Somatic ATRX mutations are seen in PCC/PGL To determine the frequency of somatic ATRX mutations in PCC/PGL, we sequenced the ATRX coding region in two validation sets of FFPE PCC/PGL using amplicon sequencing to a mean depth of coverage of 1,430 × . Validation set 1 contains PCC/PGL from 52 patients with known inherited mutation status; validation set 2 contains tumours from 51 patients without clinical genetic testing ( Supplementary Tables 3 and 4 ). We followed a strict filtering algorithm for variant calling including removing variants with MAF>0.1% in 1,000 genomes and/or ESP6500, with read depth <50 or segmental duplication >80%. ATRX variants were called mutations if the variant was a stop gain variant, insertion or deletion, or missense variant located within a known functional domain and called deleterious in three in silico prediction callers (SIFT [22] , POLYPHEN2 (ref. 23 ) and MutationTaster [24] ). In validation sets 1 and 2, we found 11.5% of tumours (6/52) and 13.7% of tumours (7/51), respectively, had somatic mutations in ATRX ( Table 1 ). The overall somatic mutation rate was 12.6%. Two tumours had two nonsynonymous alterations that passed the filtering algorithm as described in the Methods section. Both tumours are from male patients, and because ATRX is on the X chromosome, this finding implies the mutations are in cis . In both tumours, the two mutations are both within the helicase domain of ATRX , and we hypothesize that the combination of the nonsynonymous variants disrupts the function of this domain. In validation set 1 with clinical annotation, five of six tumours with somatic ATRX variants were clinically aggressive ( Table 1 and Supplementary Table 3 ). Tumours without mutations were tested for intragenic deletions by multiplex ligation-dependent probe amplification (MLPA) and none were found. These data confirm that ATRX is a frequently somatically altered gene in PCC/PGL. Table 1 Somatic Mutations in ATRX. Full size table ATRX heterodimerizes with a protein partner DAXX as part of the chromatin remodelling complex. Mutations in both genes are seen in PNETs; however, rare to no DAXX mutations are reported in neuroblastomas and gliomas [20] , [21] , [25] , [26] , [27] . We sequenced DAXX in PCC/PGL to determine if somatic mutations were present. No somatic DAXX mutations were observed in our WES of the discovery set of 21 PCC/PGL or in an independent validation set of 58 PCC/PGL by Sanger sequencing. ALT is seen in a subset of PCC/PGL The majority of cancers with somatic ATRX mutations are associated with alternative lengthening of telomeres (ALT) as a mechanism for preventing senescence. [28] , [29] To determine if PCC/PGL with somatic ATRX variants showed ALT, we performed telomere fluorescence in situ hybridization (FISH) on 22 FFPE PCC/PGL, six of which had somatic ATRX mutations ( Fig. 1 and Supplementary Tables 2–4 ). Four of the six tumours with somatic ATRX mutations showed ALT, and all four also had inherited SDHB mutations. Two tumours with somatic ATRX variants did not demonstrate ALT by this assay, suggesting the somatic mutation disrupts an alternative function of ATRX. In total, 27% of PCC/PGL (6 of the 22, 4 with ATRX mutations and 2 without) showed ALT and all were from tumours with clinically aggressive features. Two tumours with ALT had no identified somatic ATRX mutation, indicating additional genomic defects may account for elongated telomeres in some tumours. We found that 12.6% of PCC/PGL examined had somatic ATRX mutations, of which 31% have truncating mutations and 69% have missense mutations classified as deleterious based on strict criteria of being located in a known functional domain and deleterious in three in silico prediction callers. ATRX mutations are known to play a role in human disease. Germline mutations lead to X-linked alpha thalassemia mental retardation syndrome; somatic mutations are implicated as drivers in several non-epithelial cancer types including PNETs, neuroblastomas and gliomas [20] , [21] , [25] , [26] , [30] . ATRX is a large gene of ~300 kb on the X chromosome and a member of the SWI/SNF family of chromatin remodelers, which play a role in telomere maintenance and chromosome integrity [31] . ATRX has several binding partners involved in epigenetic regulation including DAXX, which acts as a chaperone to bring histone H3.3 to telomeric and pericentric regions [32] , [33] . In non-functional PNETs, somatic ATRX and DAXX mutations are common (43%) and mutually exclusive with 25% having DAXX and 17.6% having ATRX mutations [20] . We identified no somatic DAXX mutations in PCC/PGL. However, not all neuroendocrine-related tumours carry DAXX mutations. Neuroblastomas, which have somatic ATRX mutations or intragenic deletions in 9–33% of tumours, have not been demonstrated to have any DAXX mutations [21] , [25] . Furthermore, gliomas have somatic ATRX mutations in 30–58% of tumours, yet DAXX mutations are rarely, if ever, observed [26] , [27] . Preventing senescence is a hallmark of cancer cells, and most cancers have increased expression of telomerase to maintain the telomeres. However, at least 10–15% of cancers have an alternative mechanism for lengthening of telomeres (ALT) thought to involve homologous recombination. We performed telomere FISH assay for ALT on six PCC/PGL with somatic ATRX mutations and on 16 PCC/PGL without somatic ATRX mutations. Four of the 6 (67%) samples with somatic ATRX mutations showed ALT and only 2 of 16 (12.5%) samples without ATRX mutations showed ALT. Although most human cancers and cell lines with ATRX mutations have associated ALT, not all of them have demonstrated ALT as reported in multiple published studies [27] , [29] , [34] , suggesting that some mutations may disrupt alternative functions of ATRX. Currently, ATRX function is not completely understood and cellular roles beyond ALT have been described. ATRX promotes alpha globin gene expression by reducing macroH2A deposition at the alpha globin locus [35] , and promotes transcriptional repression of TERRA, the telomere RNA transcript [36] . Thus, it is possible that some ATRX mutations disrupt a function of the ATRX protein other than ALT. Other epigenetic alterations are known to exist in PCC/PGL. Studies examining the methylome suggest that PCC/PGL from patients with germline SDHx and VHL mutations are hypermethylated compared with tumours with NF1 or RET mutations, and the highest rates of methylation are in SDHB -associated tumours [37] , [38] . Mutations in SDHx genes lead to elevated levels of succinate, postulated to cause hypermethylation by inhibiting 2-oxoglutarate-dependent histone and DNA demethylase enzymes [38] , [39] . Perhaps further epigenetic dysregulation in these tumours is occurring through additional somatic mutations in genes such as ATRX , as seen in gliomas with co-occurrence of ATRX mutations and IDH mutations leading to increased alpha-ketoglutarate, postulated to cause hypermethylation through the same mechanism as succinate [26] . In PNETs, initial analysis found that tumours with somatic ATRX (or heterodimerizing partner DAXX ) mutations were associated with better prognosis [20] . However, a recent study, analysing two larger cohorts found that tumours with somatic ATRX (or DAXX ) mutations (implied by negative immunohistochemical staining) were associated with worse prognosis than tumours without a mutation [40] . Our sample set of PCC/PGL with ATRX mutations is too small to draw definitive conclusions regarding prognosis, especially given the long latency in this disease. Nevertheless, it is interesting to note that of the tumours with known clinical genetic testing, most tumours with somatic ATRX mutations also have inherited SDHx mutations. This study is the first to our knowledge to use WES in matched tumour and germline pairs to identify somatic alterations in PCC/PGL. We identified somatic ATRX mutations in 12.6% of PCC/PGL. Although our sample set of PCC/PGL with ATRX variants is too small to identify statistically significant associations, many had clinically aggressive features, inherited SDHx mutations and ALT, suggesting an interaction between the somatic and inherited genomes in solid cancers, which needs to be investigated further. Future work needs to be done to clarify the role of ATRX mutations on epigenetic regulation in PCC/PGL and to identify other somatic alterations involved in PCC/PGL tumorigenesis and malignant transformation. Samples This study was performed under an IRB approved protocol at the University of Pennsylvania with patients providing signed informed consent. A discovery set of 21 PCC/PGL were selected to represent clinically benign and clinically aggressive tumours. The clinical data from all subjects are described in Supplementary Table 1 . Fresh-frozen PCC/PGL were sectioned and stained with hematoxylin and eosin to ensure sections of over 70% tumour are used for DNA extraction. DNA was extracted from tumour tissue using Qiagen AllPrep kits. Germline DNA from blood or saliva was extracted using standard protocols in the laboratory. All DNA was quantitated with a Qubit. To ensure high-quality genomic DNA, the A260/280 ratio was measured on a Nanodrop and DNA was run on a 1% agarose gel. Two separate validation sets of DNA from FFPE PCC/PGL were used. The tumour samples in the validation set were collected from subjects with PCC/PGL who had surgery at the University of Pennsylvania or the University of Michigan. The University of Michigan samples were from the Cancer Genetics Registry (CGN, HUM00043430) and Michigan Endocrine Oncology Repository (MEOR, HUM00024461). Validation set 1 includes samples from 52 patients with known clinical germline testing results. Validation set 2 was derived from 51 patients who did not have clinical genetic testing. In validation set 1, 31 of 52 subjects had known inherited mutations in PCC/PGL susceptibility genes (9 SDHB , 8 SDHD , 4 SDHC , 2 RET , 6 NF1 and 2 VHL ), whereas 21 other subjects who had clinical genetic testing had no identified germline mutation (considered sporadic tumours). Massively parallel sequencing We performed WES of fresh-frozen tumour and matched germline DNA using Illumina TruSeq Sample Prep kits for library preparation and Agilent SureSelect Human All Exon v3 kit for exome enrichment. In brief, for each matched germline and tumor sample, 1 μg of DNA was sheared with a Covaris sonicator to fragments of 200 base pairs (bp). Samples were A-tailed and ligated with adaptor-embedded indexes to allow for multiplexing. DNA quality and fragment size were measured with an Agilent 2100 Bioanalyzer and concentration measured with a Qubit. Samples were pooled and sequenced on the Illumina HiSeq2000 in the Penn Functional Genomics Core , with an average of six germline exomes and three tumour exomes per lane (each lane producing 200 million clusters of 100 bp paired-end reads). Alignment and variant calling Raw sequencing data were aligned and mapped to the reference genome hg19 using the Burrows–Wheeler Aligner [41] . Duplicate reads were removed, as well as reads that map to more than one location. Genome Analysis Toolkit (GATK) was used for single-nucleotide variant (SNV) calling and for identifying small insertions and deletions in tumour and matched germline WES data [42] . Variants found in common between the matched germline and tumour DNA were removed to keep only variants unique to the tumour (somatic variants). During the analysis stage, phred scores and mapping quality scores were set to 30 allowing for 99.9% base-calling accuracy and read mapping accuracy, respectively. Variants with read depth <20 were removed. Annotation Variants were annotated using ANNOVAR to call variants as frameshift indel, non-frameshift indel, stop gain, stop loss, synonymous, nonsynonymous and splicing (intronic and exonic) [43] . ANNOVAR also annotates single-nucleotide variants using SIFT, Polyphen2 and MutationTaster to make predictions about pathogenicity and PhyloP and +GERP to make predictions about conservation [22] , [23] , [24] , [43] , [44] , [45] . Variants were removed if the alternate allele frequency was less than 5%, if the segmental duplication was above 80% or the minor allele frequency (MAF) was above 0.1% in EVS6500 and/or 1,000 genomes. Synonymous variants were considered benign and removed. Amplicon sequencing of ATRX DNA from FFPE PCC/PGL from the validation sets were used to test for somatic ATRX variants by multiplex amplicon sequencing. Primers were designed across the coding region of ATRX and modified with adaptors to allow for subsequent sequencing on the Illumina Miseq. One hundred and seven primer sets spanned the coding region and were divided into seven PCR primer pools. Each tumour sample was PCR amplified with all seven primer pools. Standard PCR protocol was used with the following parameters: 5 cycles at each of the following annealing temperature 68, 63, 60 and 58 °C followed by 15 cycles at annealing temperature of 55 °C. The seven reactions per sample were combined and purified using AMPure XP beads (Agencourt). Samples were diluted 1:20. Two microliters of the purified and diluted samples were used as template for a second round of PCR using indexed primers from Illumina TruSeq Custom Amplicon Index Kit (Dual index) (FC-130–1003) to allow for multiplexing. Standard PCR conditions were used for the second round of PCR including five cycles at each of the following annealing temperatures of 68 °C and then 62 °C. PCR products were again purified with AMPure XP beads (Agencourt) and quantified using a Qubit. Samples were multiplexed equimolar and run on the Illumina MiSeq. Raw sequencing data were analysed using the pipeline described in Daber et al . [46] . Only variants with MAF <0.1% in both EVS6500 and 1,000 genomes and a read depth of at least 50 were considered for analysis. Only nonsense, frameshift, splice site and missense variants located in a functional domain of the protein and considered damaging in at least three in silico pathogenicity predication programs (described above) were called somatic mutations. Sanger sequencing of DAXX DNA from FFPE PCC/PGL from the validation sets were used to test for somatic DAXX variants by Sanger sequencing. Primers were designed across the entire coding region of DAXX . Primer sequences are provided in Supplementary Table 5 . Standard PCR protocol was used with 35 cycles at primer-specific annealing temperatures given in Supplementary Table 5 . PCR products were cleaned up using exonuclease reactions and sequenced using BigDye Terminator v3.1 (Applied Biosystems) and run on an ABI Prism 3130 × l Genetic Analyzer. Immunohistochemistry Immunohistochemistry (IHC) was done to confirm the effect of the mutations on the ATRX protein in the FFPE tumour tissue. Slides were deparaffinized in xylene and rehydrated in a graded ethanol series. Heat‐induced antigen retrieval was performed in a steamer using citrate buffer (pH 6.0) (Vector Laboratories) for 30 min followed by 10 min of cooling. Endogenous peroxidase was blocked for 10 min with dual endogenous enzyme‐blocking reagent (Dako). Serial sections were then incubated with primary antibody; anti‐ATRX (1:400) (Sigma‐Aldrich; HPA001906) and anti‐DAXX (1:75) (Sigma‐Aldrich; HPA008736) for 1 h at room temperature. The sections were then incubated for 30 min with secondary antibody (Leica Microsystems) followed by detection with 3,3′‐Diaminobenzidine (Sigma‐Aldrich) for 8 min. Sections were washed with phosphate‐buffered saline with 0.1% Tween‐20. Finally, sections were counterstained with hematoxylin, subsequently rehydrated in a graded ethanol series and mounted. Only nuclear labelling of either protein in tumour cells was considered positive. Endothelial cells on each section served as internal controls. Telomere FISH Mutations in ATRX have been associated with ALT [28] . To examine the ALT phenotype, we performed telomere-specific FISH per protocol by Heaphy et al . [28] with some modifications. Slides were deparaffinized in xylene and rehydrated in a graded ethanol series. Antigen retrieval was performed by boiling slides in 100 mM Tris with 50 mM EDTA for 10 min and allowed to cool for 5 min at room temperature. Slides were then treated with 0.5 mg per ml of protease type VIII (Sigma) treatment for 1 min at room temperature. Wash buffer was prepared (70% formamide, 24% ddH 2 O, 10 nM Tris pH 7.5 and 0.5% blocking solution (Roche)). Slides were probed using a peptide nucleic acid (PNA) FISH probe (1:100 in PNA wash buffer) (Panagene; F1002-5 TelC-Cy3) by denaturing at 83 °C for 4 min and incubating at room temperature for 2 h. Slides were washed twice in PNA wash buffer for 30 min and counterstained with DAPI (1:750) (Invitrogen). After hydration in a graded ethanol series, slides were mounted with Vectashield antifade (Vectalabs) and imaged on a Nikon 80i/ fluorescent microscope using a Qimaging retiga SRV camera. Positive cells were counted across ten 20 × fields per section. Multiplex ligation-dependent probe amplification (MLPA) MLPA was performed according to manufacturer’s conditions using a commercial kit (MRC Holland; P013-100R) and analysed using Coffalyser.Net (MRC Holland; version 140429.1057). How to cite this article: Fishbein L. et al . Whole-exome sequencing identifies somatic ATRX mutations in pheochromocytomas and paragangliomas. Nat. Commun. 6:6140 doi: 10.1038/ncomms7140 (2015). Accession codes: Sequence data for the PCC/PGL have been deposited in GenBank/EMBL/DDBJ Sequence Read Archive (SRA) under the accession code SRP050479 .